TNF-α blockade induces IL-10 expression in human CD4+ T cells IL-17+ CD4+ T (Th17) cells contribute to the pathogenesis of several human inflammatory diseases. Here we demonstrate that TNF inhibitor (TNFi) drugs induce the anti-inflammatory cytokine IL-10 in CD4+ T cells including IL-17+ CD4+ T cells. TNFi-mediated induction of IL-10 in IL-17+ CD4+ T cells is Treg-/Foxp3-independent, requires IL-10 and is overcome by IL-1β. TNFi-exposed IL-17+ CD4+ T cells are molecularly and functionally distinct, with a unique gene signature characterized by expression of IL10 and IKZF3 (encoding Aiolos). We show that Aiolos binds conserved regions in the IL10 locus in IL-17+ CD4+ T cells. Furthermore, IKZF3 and IL10 expression levels correlate in primary CD4+ T cells and Aiolos overexpression is sufficient to drive IL10 in these cells. Our data demonstrate that TNF-α blockade induces IL-10 in CD4+ T cells including Th17 cells and suggest a role for the transcription factor Aiolos in the regulation of IL-10 in CD4+ T cells. IL-17-producing CD4+ T cells (often referred to as Th17 cells) are considered critical contributors to the pathogenesis of several human inflammatory diseases [1] . IL-17+ CD4+ T cells have potent pro-inflammatory effects, are enriched at sites of inflammation and correlate with markers of disease activity in inflammatory diseases [1] , [2] , [3] . Results from recent clinical trials using IL-17 blocking drugs further underscore the pathogenic role of Th17 cells in human inflammatory diseases [4] . The polarizing conditions for Th17 cell differentiation in vitro are increasingly well defined; however, accumulating evidence indicates that once differentiated, CD4+ effector T cell lineages display a considerable degree of plasticity and diversity [5] , [6] . Human CD4+ T cells can co-express IL-17 and IFN-γ, particularly at sites of inflammation [3] , [7] . Foxp3+ CD4+ regulatory T cells (Tregs) can gain IL-17 expression and cells co-expressing RORγt and Foxp3 can be detected in vivo [8] . Furthermore, mouse models revealed that Th17 cells can gain expression of the anti-inflammatory cytokine IL-10 and become non-pathogenic when stimulated in the presence of IL-6 and TGF-β, while stimulation in the presence of IL-23 maintains their pathogenicity [9] , [10] . The small intestine was shown to play a key role in the induction of immunosuppressive IL-17+IL-10+ CD4+ T cells [11] . A recent study in humans demonstrated that depending on the pathogen encountered ( Candida albicans versus Staphylococcus aureus ), Th17 cells can co-express significant amounts of IFN-γ or IL-10, respectively [12] . The ability to co-express IL-10 indicates that Th17 cells have an intrinsic ability to self-regulate. Understanding how IL-10 induction in pro-inflammatory Th17 cells is regulated is therefore of considerable immunological and clinical interest. TNF-inhibitor (TNFi) drugs have been used to treat millions of patients worldwide, thereby transforming the treatment of immune-mediated inflammatory diseases. Here we use treatment with TNFi drugs as a model system to investigate whether the resulting changes in the pro-inflammatory environment affect the function and phenotype of human IL-17+ CD4+ T cells. We demonstrate that a counterintuitive rise in the percentage of IL-17+ CD4+ T cells following TNFi therapy may be explained by the acquisition of anti-inflammatory properties by these typically pathogenic cells. We show that TNFi-exposed IL-17+ CD4+ T cells express high levels of IL-10, which is Treg-/Foxp3-independent and relies on an IL-10 positive feedback loop, and is overcome by the addition of the pro-inflammatory cytokine IL-1β. Interestingly, TNFi-exposed IL-17+ CD4+ T cells are functionally and molecularly distinct, with increased expression of IKZF3 encoding the transcription factor Aiolos, which binds conserved regions in the IL10 locus in IL-17+ CD4+ T cells. Our data provide evidence to suggest that the transcription factor Aiolos may be a regulator of IL-10 expression in human CD4+ T cells. TNFi drugs increase IL-17+ and IL-10+ CD4+ T cells We have previously shown that patients with rheumatoid arthritis (RA) have an increased percentage of IL-17+IFN-γ- CD4+ T cells in their peripheral blood compared with healthy controls [3] . When patients with RA were separated on the basis of their treatment regimen, that is, disease-modifying anti-rheumatic drug (DMARD) therapy or TNF-inhibitor (TNFi) therapy, a significantly higher percentage of peripheral IL-17+ CD4+ T cells was observed in patients receiving TNFi therapy (median (IQR) 1.4% (0.8–2.4)) relative to those receiving DMARD (0.6% (0.4–1.1)) or healthy controls (0.4% (0.3–0.7)) ( Fig. 1a ; gating strategy shown in Supplementary Fig. 1 ). The increase in the percentage of IL-17+ CD4+ T cells was not related to differences in clinical parameters of disease (disease activity score (DAS28), erythrocyte sedimentation rate or C-reactive protein) or patient characteristics (rheumatoid factor positivity, age and gender) between the two treatment groups ( Supplementary Fig. 2 ). Interestingly, we also observed a concurrent increase in the percentage of CD4+ T cells expressing the anti-inflammatory cytokine IL-10 in the peripheral blood of TNFi-treated patients ( Fig. 1b ). 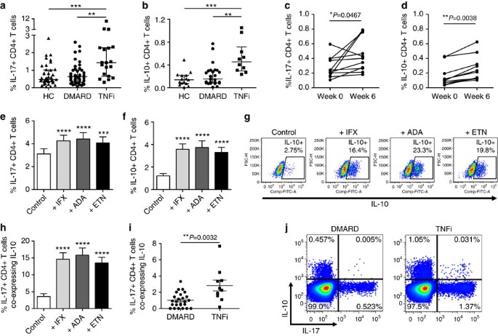Figure 1:TNFi drugs increase the percentages of IL-17+ and IL-10+ CD4+ T cellsin vivoandin vitro. Percentages (median with interquartile range) of IL-17+ (a) and IL-10+ (b) cells within the total peripheral CD4+ T cell population were analysed in healthy controls (HC,n=15–41), and patients with RA on DMARD (n=25–42) versus TNFi therapy (n=10–19). Data analysed by ANOVA (Kruskal–Wallis test) followed by Dunn’s Multiple Comparison Test. **P<0.01, ***P<0.001. Percentages of IL-17+ (c) and IL-10+ (d) cells within peripheral blood CD4+ T cells of patients with spondyloarthritis (n=11) before (week 0) and 6 weeks after (week 6) the start of TNFi therapy (analysed by Wilcoxon matched-pairs signed rank test or pairedt-test). (e–h) CD4+ T cells and CD14+ monocytes from healthy controls were co-cultured with anti-CD3 mAb (Control) with or without 1 μg ml−1of infliximab (IFX), adalimumab (ADA) or etanercept (ETN), followed by PMA/ionomycin restimulation on day 3. Percentages of IL-17+ (e) and IL-10+ (f) cells within total CD4+ T cells are shown (mean±s.e.m.,n=15). Representative dot plots (g) and cumulative data (h) of the same cultures showing the percentage of IL-17+ CD4+ T cells co-expressing IL-10. Data analysed by repeated measures ANOVA followed by Bonferroni’s Multiple Comparison test. ***P<0.001, ****P<0.0001 relative to control. Cumulative data (i) and representative dot plots (j) showing the percentage of IL-17+ CD4+ T cells co-expressing IL-10 in the peripheral blood of patients with RA on DMARD (n=25) or TNFi therapy (n=10). Data shown as mean±s.e.m., analysed by Mann–Whitney test. Figure 1: TNFi drugs increase the percentages of IL-17+ and IL-10+ CD4+ T cells in vivo and in vitro . Percentages (median with interquartile range) of IL-17+ ( a ) and IL-10+ ( b ) cells within the total peripheral CD4+ T cell population were analysed in healthy controls (HC, n =15–41), and patients with RA on DMARD ( n =25–42) versus TNFi therapy ( n =10–19). Data analysed by ANOVA (Kruskal–Wallis test) followed by Dunn’s Multiple Comparison Test. ** P <0.01, *** P <0.001. Percentages of IL-17+ ( c ) and IL-10+ ( d ) cells within peripheral blood CD4+ T cells of patients with spondyloarthritis ( n =11) before (week 0) and 6 weeks after (week 6) the start of TNFi therapy (analysed by Wilcoxon matched-pairs signed rank test or paired t -test). ( e – h ) CD4+ T cells and CD14+ monocytes from healthy controls were co-cultured with anti-CD3 mAb (Control) with or without 1 μg ml −1 of infliximab (IFX), adalimumab (ADA) or etanercept (ETN), followed by PMA/ionomycin restimulation on day 3. Percentages of IL-17+ ( e ) and IL-10+ ( f ) cells within total CD4+ T cells are shown (mean±s.e.m., n =15). Representative dot plots ( g ) and cumulative data ( h ) of the same cultures showing the percentage of IL-17+ CD4+ T cells co-expressing IL-10. Data analysed by repeated measures ANOVA followed by Bonferroni’s Multiple Comparison test. *** P <0.001, **** P <0.0001 relative to control. Cumulative data ( i ) and representative dot plots ( j ) showing the percentage of IL-17+ CD4+ T cells co-expressing IL-10 in the peripheral blood of patients with RA on DMARD ( n =25) or TNFi therapy ( n =10). Data shown as mean±s.e.m., analysed by Mann–Whitney test. Full size image In order to determine whether the increase in IL-17+ and IL-10+ CD4+ T cells was a drug-induced effect, we measured IL-17+ and IL-10+ CD4+ T cell frequencies longitudinally in cryopreserved peripheral blood mononuclear cells (PBMC) from a cohort of patients with peripheral spondyloarthritis pre/post TNFi therapy [13] . Significantly higher levels of IL-17+ and IL-10+ CD4+ T cells were detected in samples collected 6 weeks after the start of TNFi therapy compared with samples taken at the start of therapy ( Fig. 1c,d ). These data indicate that TNFi therapy leads to an increase in the percentages of both IL-17+ and IL-10+ CD4+ T cells in peripheral blood in vivo . To further examine the increase in IL-17+ and IL-10+ CD4+ T cells, in vitro co-cultures of CD4+ T cells and autologous CD14+ monocytes from healthy donors in the presence of anti-CD3 mAb were set up, a system previously shown by our group to induce IL-17 responses in human memory CD4+ T cells [14] , [15] . Cells were cultured in the absence or presence of 1 μg ml −1 of infliximab (IFX), adalimumab (ADA) or etanercept (ETN), TNFi drugs routinely used in clinical practice. After 3 days, cells were pulsed with PMA/ionomycin in the presence of GolgiStop and stained intracellularly for the presence of cytokines. In vitro addition of each of the three TNFi drugs led to a significant increase in the percentages of both IL-17+ and IL-10+ CD4+ T cells relative to control-treated cells ( Fig. 1e,f ). Interestingly, when added in vitro, all three TNFi drugs (IFX, ADA and ETN) also stimulated a significant proportion of IL-17+ CD4+ T cells to co-express IL-10 (on average 15%) ( Fig. 1g,h ), suggesting that in the presence of TNFi drugs Th17 cells acquire anti-inflammatory properties. Addition of non-specific IgG1 antibodies did not increase the percentage of IL-17+ CD4+ T cells co-expressing IL-10, indicating that this was a drug-specific effect ( Supplementary Fig. 3 ). Cross-sectional analysis of patients with RA treated with TNFi therapy also revealed a significant increase in IL-17+ CD4+ T cells co-expressing IL-10 when compared with patients receiving DMARD therapy ( Fig. 1i,j ). These data indicate that the counterintuitive increase in IL-17+ CD4+ T cells upon treatment with TNFi drugs may be counterbalanced by the acquisition of an anti-inflammatory potential by these cells. IL-10 promotes and IL-1β counteracts TNFi-induced IL-10 Having demonstrated that TNFi drugs can stimulate the expression of IL-10 in otherwise inflammatory IL-17+ CD4+ T cells, we next sought to identify the cellular mechanism that promotes this response. It has been suggested previously that the presence of TNF-α can inhibit CD4+CD25+ Treg function and that TNFi drugs enhance Treg-mediated suppression [16] , [17] . To determine whether the presence of Tregs was critical for the induction of IL-10 expression in IL-17+ CD4+ T cells, we separated PBMC into total CD4+ T cells and Treg-depleted responder cells (CD4+CD25- T cells). Irrespective of the presence or absence of CD4+CD25+ Tregs, the proportion of IL-17+ T cells co-expressing IL-10 was increased in the presence of adalimumab ( Fig. 2a ; Supplementary Fig. 4a ). IL-10 co-expression by IL-17+ CD4+ T cells occurred within the memory CD4+ T cell population, suggesting that it did not involve inducible Treg generation from naive CD4+ T cells ( Supplementary Fig. 4a,b ). Furthermore, we found that the majority (>80%) of IL-17+ T cells were Foxp3−, while only a very small percentage (on average <5%) of the total Foxp3+ T cells expressed IL-17 or IL-10 in either TNFi-exposed or control conditions ( Fig. 2b and Supplementary Fig. 4c,d ). Finally, no increase in the percentage of Foxp3+ cells within the CD4+ T cell population as a whole or within the IL-17+IL-10+ CD4+ T cells was observed upon treatment with TNFi drugs ( Fig. 2c,d ). Together, these data indicate that the TNFi-mediated induction of IL-10 co-expressing IL-17+ CD4+ T cells occurs independently of Tregs and Foxp3. 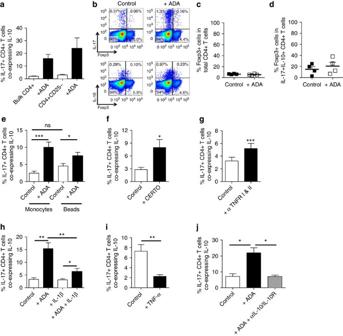Figure 2: Dissecting the cellular mechanisms underlying the TNFi-mediated induction of IL-10 co-expression by IL-17+ CD4+ T cells. (a) PBMC were separated into bulk CD4+ T cells or Treg-depleted CD4+CD25- T cells (n=3) and co-cultured with monocytes with anti-CD3 mAb +/- ADA for 3 days. Cells were stimulated with PMA/ionomycin/GolgiStop and stained for IL-17 and IL-10. (b–d) Bulk CD4+ T cells were cultured with monocytes and anti-CD3 mAb in the absence or presence of ADA for 3 days followed by stimulation and staining for IL-17, IL-10 and Foxp3. Representative dot plots (b) and the percentage of Foxp3+ cells within total CD4+ T cells (c) or within IL-10+ IL-17+ CD4+ T cells are shown (d) (median±IQR,n=4). (e) CD4+ T cells were cultured for 3 days without/with ADA, with either anti-CD3 and CD14+ monocytes or anti-CD3/CD28 microbeads (n=12). The percentage of IL-17+ CD4+ T cells co-expressing IL-10 is shown. (f) CD4+ T cells and monocytes were co-cultured with anti-CD3 mAb with/without 1 μg/ml certolizumab (CERTO,n=7). (g) Co-cultures were set up in the absence/presence of blocking Abs against TNFRI and II (n=8). (h) Co-cultures were set up with/without ADA in the absence or presence of hrIL-1β (n=9). (i,j) Memory enriched CD4+ T cells were co-cultured with CD14+ monocytes and anti-CD3 in the absence or presence of TNF-α (n=8) (i) or in the absence or presence of adalimumab ± neutralizing Abs against IL-10 and IL-10R (n=6) (j). All data are shown as mean±s.e.m. Data were analysed by repeated measures ANOVA followed by Bonferroni’s or Dunn’s Multiple Comparison test, or by pairedt-test or Wilcoxon matched-pairs signed-rank test. *P<0.05; **P<0.01; ***P<0.001. Figure 2: Dissecting the cellular mechanisms underlying the TNFi-mediated induction of IL-10 co-expression by IL-17+ CD4+ T cells. ( a ) PBMC were separated into bulk CD4+ T cells or Treg-depleted CD4+CD25- T cells ( n =3) and co-cultured with monocytes with anti-CD3 mAb +/- ADA for 3 days. Cells were stimulated with PMA/ionomycin/GolgiStop and stained for IL-17 and IL-10. ( b – d ) Bulk CD4+ T cells were cultured with monocytes and anti-CD3 mAb in the absence or presence of ADA for 3 days followed by stimulation and staining for IL-17, IL-10 and Foxp3. Representative dot plots ( b ) and the percentage of Foxp3+ cells within total CD4+ T cells ( c ) or within IL-10+ IL-17+ CD4+ T cells are shown ( d ) (median±IQR, n =4). ( e ) CD4+ T cells were cultured for 3 days without/with ADA, with either anti-CD3 and CD14+ monocytes or anti-CD3/CD28 microbeads ( n =12). The percentage of IL-17+ CD4+ T cells co-expressing IL-10 is shown. ( f ) CD4+ T cells and monocytes were co-cultured with anti-CD3 mAb with/without 1 μg/ml certolizumab (CERTO, n =7). ( g ) Co-cultures were set up in the absence/presence of blocking Abs against TNFRI and II ( n =8). ( h ) Co-cultures were set up with/without ADA in the absence or presence of hrIL-1β ( n =9). ( i , j ) Memory enriched CD4+ T cells were co-cultured with CD14+ monocytes and anti-CD3 in the absence or presence of TNF-α ( n =8) ( i ) or in the absence or presence of adalimumab ± neutralizing Abs against IL-10 and IL-10R ( n =6) ( j ). All data are shown as mean±s.e.m. Data were analysed by repeated measures ANOVA followed by Bonferroni’s or Dunn’s Multiple Comparison test, or by paired t -test or Wilcoxon matched-pairs signed-rank test. * P <0.05; ** P <0.01; *** P <0.001. Full size image To examine the importance of monocytes in the induction of IL-10 co-expression by IL-17+ CD4+ T cells, co-cultures were set up with either monocytes and anti-CD3 mAb or with anti-CD3/CD28 Ab-coated beads in the presence or absence of adalimumab. As shown before, the addition of TNFi drugs in the presence of monocytes led to a strong increase in the percentage of IL-17+ CD4+ T cells co-expressing IL-10; however, there was also a significant increase in IL-17+ CD4+ T cells co-expressing IL-10 in the presence of anti-CD3/CD28 beads ( Fig. 2e ), albeit to a lesser degree, suggesting that this process is not entirely monocyte-dependent. It should however be noted that in the presence of beads the total percentage of IL-17+ CD4+ T cells was considerably reduced ( Supplementary Fig. 4e and ref. 14 ), highlighting the importance of monocytes for the induction of IL-17 responses in human CD4+ T cells. Reduced induction of IL-10 co-expression by IL-17+ CD4+ T cells was observed when CD14-depleted accessory cells were added instead of CD14+ monocytes ( Supplementary Fig. 4f ) or when cell-contact between monocytes and T cells was prevented ( Supplementary Fig. 4g ). Together, these data suggest that although the presence of monocytes is not an absolute requirement for IL-10 expression in IL-17+ CD4+ T cells, monocytes do potentiate this effect. The three TNF inhibitors used thus far (infliximab, adalimumab and etanercept) all contain Fc domains, raising the possibility that binding or signalling through the FcγR might be involved in driving the responses observed. The induction of IL-10 expression in IL-17+ CD4+ T cells was however found to be FcγR-independent, as shown by the addition of certolizumab, a PEGylated Fab' fragment of humanized anti-TNF-α mAb ( Fig. 2f ) and by the addition of FcγR-blocking reagent ( Supplementary Fig. 4h ). Instead, the increase in IL-10 co-expression in IL-17+ CD4+ T cells appeared to be due to a loss of TNF-α signalling through its receptor, as addition of blocking Abs to TNFRI and II also significantly increased the percentage of IL-17+ CD4+ T cells co-expressing IL-10 ( Fig. 2g ). Interestingly, the addition of hrIL-1β, a potent pro-inflammatory cytokine, led to a significant reduction in TNFi-induced IL-10 co-expression in IL-17+ CD4+ T cells ( Fig. 2h ). Furthermore, addition of hrTNF-α significantly reduced the percentage of IL-17+ CD4+ T cells co-expressing IL-10 in memory CD4+ T cells ( Fig. 2i ). Mechanistically, the co-expression of IL-10 by IL-17+ CD4+ T cells was found to rely on an IL-10 positive feedback loop as addition of blocking antibodies to IL-10 and IL-10R decreased the induction of IL-17+ CD4+ T cells co-expressing IL-10 ( Fig. 2j ). Together, these data indicate that the induction of IL-10 co-expression in human IL-17+ CD4+ T cells is IL-10-dependent, and can be overcome by inflammatory cytokines. TNFi-exposed IL-17+ CD4+ T cells are functionally distinct Next we examined the functional consequences of TNFi exposure on IL-17+ CD4+ T cells. Control and TNFi-exposed IL-17+ CD4+ T cells were sorted using a cytokine secretion assay ( Supplementary Fig. 5 ) and cultured overnight. Supernatants from TNFi-exposed IL-17+ CD4+ T cells contained significantly increased levels of IL-10, while maintaining high levels of IL-17 and IFN-γ ( Fig. 3a ). These data suggest that TNFi-exposed IL-17+ CD4+ T cells acquire regulatory potential rather than lose their inflammatory capacity. 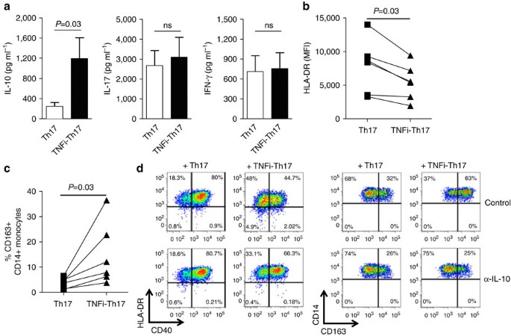Figure 3: TNFi-exposed Th17 cells are functionally distinct. CD4+ T cells and monocytes were co-cultured with anti-CD3 mAb in the absence or presence of adalimumab for 3 days. (a) Sorted IL-17+CD4+ T cells (100,000 cells per well) from both conditions were cultured overnight and cell culture supernatants collected to test for the presence of the indicated cytokines (mean±s.e.m.,n=6). (b,c) Sorted control-treated (Th17) or TNFi-exposed (TNFi-Th17) IL-17+ CD4+ T cells were added to autologous or allogeneic CD14+ monocytes at a 1:2 ratio and monocyte phenotype was assessed after 20 h by flow cytometry. Graphs show the expression of HLA-DR (MFI) (b) and the percentage of CD163+CD14+ monocytes (c) (n=6). (d) Sorted Th17 cells were added to monocytes in the absence or presence of neutralizing anti-IL-10 mAb (10 μg ml−1) and monocyte phenotype was measured; one of two experiments shown. Data in (a–c) were analysed by Wilcoxon matched-pairs signed-rank test. Figure 3: TNFi-exposed Th17 cells are functionally distinct. CD4+ T cells and monocytes were co-cultured with anti-CD3 mAb in the absence or presence of adalimumab for 3 days. ( a ) Sorted IL-17+CD4+ T cells (100,000 cells per well) from both conditions were cultured overnight and cell culture supernatants collected to test for the presence of the indicated cytokines (mean±s.e.m., n =6). ( b , c ) Sorted control-treated (Th17) or TNFi-exposed (TNFi-Th17) IL-17+ CD4+ T cells were added to autologous or allogeneic CD14+ monocytes at a 1:2 ratio and monocyte phenotype was assessed after 20 h by flow cytometry. Graphs show the expression of HLA-DR (MFI) ( b ) and the percentage of CD163+CD14+ monocytes ( c ) ( n =6). ( d ) Sorted Th17 cells were added to monocytes in the absence or presence of neutralizing anti-IL-10 mAb (10 μg ml −1 ) and monocyte phenotype was measured; one of two experiments shown. Data in ( a – c ) were analysed by Wilcoxon matched-pairs signed-rank test. Full size image To determine whether the increased IL-10 production by TNFi-exposed IL-17+ CD4+ T cells had functional consequences, control or TNFi-exposed IL-17+ CD4+ T cells were sorted and added to freshly isolated CD14+ monocytes. Monocyte phenotype was examined at 20 h. While control IL-17+ CD4+ T cells induced an upregulation of HLA-DR and CD40 expression on monocytes, TNFi-exposed IL-17+ CD4+ T cells were significantly reduced in this capacity ( Fig. 3b,d ). Instead, in the presence of TNFi-exposed IL-17+ CD4+ T cells, an increase was observed in the percentage of CD14+ monocytes expressing the haptoglobin/haemoglobin scavenger receptor CD163, a molecule known to be regulated by IL-10 (ref.18) [18] ; ( Fig. 3c,d ). The effect of TNFi-exposed IL-17+ CD4+ T cells on monocyte phenotype was reversed when neutralizing anti-IL-10 mAbs were added ( Fig. 3d ). Together, these data indicate that TNFi-exposed IL-17+ CD4+ T cells are functionally distinct and produce biologically active IL-10. TNFi-exposed IL-17+ CD4+ T cells are molecularly distinct Next, we performed gene expression profiling of control and TNFi-exposed IL-17+ CD4+ T cells. Analysis of nine paired samples revealed 42 differentially expressed genes when analysed at a 1% false-discovery rate (FDR) and 813 genes at a 5% FDR ( Fig. 4a ), indicating that TNFi-induced Th17 cells are molecularly distinct, with a unique gene expression profile. The fold enrichment of the top 25 upregulated genes is shown in Fig. 4b . Among these genes, we found significantly increased levels of IL10 ( P =0.000063 (paired t -test), q =0.01 (adjusted P -values using the Benjamini–Hochberg procedure) ( Fig. 4c ), confirming our flow cytometry and cytokine secretion data. No significant differences were detected in the expression of IL17A , IL17F and IFNG ( Fig. 4c ) or the transcription factors RORC , TBX21 , GATA3 and FOXP3 ( Fig. 4d ). A very small but significant increase in MAF expression was detected in TNFi-exposed IL-17+ CD4+ T cells ( Fig. 4d ), which could contribute to the increase in IL-10 expression [19] . 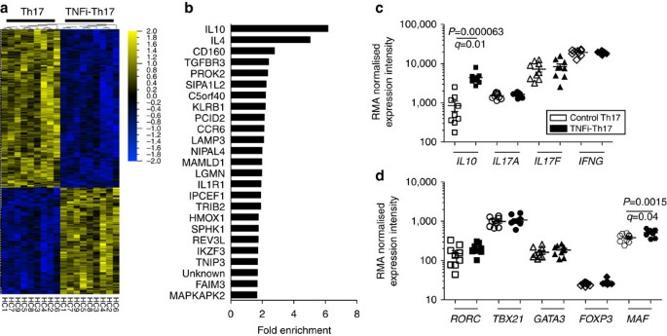Figure 4: TNFi-exposed Th17 cells are molecularly distinct. CD4+ T cells and monocytes were co-cultured with anti-CD3 mAb in the absence (Th17) or presence of adalimumab (TNFi-Th17). IL-17+ T cells were re-sorted on day 3 for gene expression profiling. (a) Heat map of differentially expressed genes (5% FDR) in control-treated versus TNFi-exposed IL-17+ CD4+ T cells. (b) The top 25 upregulated genes are shown with their average fold enrichment. (c,d) RMA normalized expression levels of indicated genes (mean±s.e.m.,n=9 independent healthy donors;q-values indicateP-values corrected for multiple testing (Benjamini–Hochberg method)). Figure 4: TNFi-exposed Th17 cells are molecularly distinct. CD4+ T cells and monocytes were co-cultured with anti-CD3 mAb in the absence (Th17) or presence of adalimumab (TNFi-Th17). IL-17+ T cells were re-sorted on day 3 for gene expression profiling. ( a ) Heat map of differentially expressed genes (5% FDR) in control-treated versus TNFi-exposed IL-17+ CD4+ T cells. ( b ) The top 25 upregulated genes are shown with their average fold enrichment. ( c , d ) RMA normalized expression levels of indicated genes (mean±s.e.m., n =9 independent healthy donors; q -values indicate P -values corrected for multiple testing (Benjamini–Hochberg method)). Full size image Correlation between IKZF3 and IL10 expression One of the genes that was most significantly upregulated at 1% FDR in TNFi-exposed IL-17+ CD4+ T cells was IKZF3 , encoding the transcription factor Aiolos ( P =0.0000071, q =0.0072) ( Fig. 5a ). IKZF3 is a member of the IKAROS family of zinc-finger domain containing transcription factors; however, other members such as IKZF1 (Ikaros), IKZF2 (Helios), IKZF4 (Eos) and IKZF5 (Pegasus) were not significantly increased ( Supplementary Fig. 6 ). The increased IKZF3 expression in TNFi-exposed IL-17+ CD4+ T cells was confirmed by real-time PCR in independent samples ( Fig. 5b ). We also analysed protein expression of Aiolos using a monoclonal anti-Aiolos Ab that recognizes the unique N-terminal part of Aiolos that is not conserved among other IKAROS family members, as confirmed by peptide blocking assay ( Supplementary Fig. 7 ). We found enhanced Aiolos expression in TNFi-exposed IL-17+ CD4+ T cells in three out of three donors by confocal imaging ( Fig. 5c,d ) and in three out of four donors by western blot analysis ( Fig. 5e,f and Supplementary Fig. 8 ). Furthermore, confocal imaging indicated that Aiolos expression was restricted to the nucleus ( Fig. 5c ). 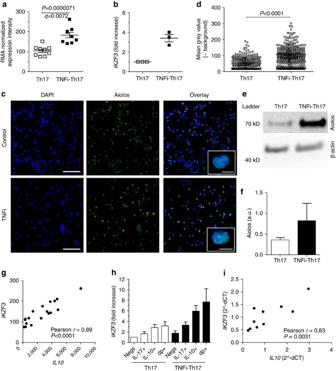Figure 5: TNFi-exposed IL-17+ CD4+ T cells express increased levels of the transcription factorIKZF3associated withIL10expression. CD4+ T cells and monocytes were co-cultured with anti-CD3 mAb in the absence or presence of adalimumab, and IL-17+ CD4+ T cells were sorted on day 3. (a) The RMA-normalized expression intensity forIKZF3is shown forn=9 paired samples (mean with s.e.m.). (b)IKZF3expression (mean with s.e.m.) was determined in three independent samples by real-time PCR, normalized toGAPDH. (c) Confocal microscopy of sorted control and TNFi-exposed IL-17+ CD4+ T cells stained for Aiolos (green). Nuclei were stained with DAPI (blue). Inserts (right) show single cells, demonstrating co-localization of Aiolos with DAPI in both conditions. Scale bars, 40 μm; 10 μm in inserts. (d) Quantification (mean grey value with 95% CI, corrected for background) of Aiolos staining per nucleus from confocal microscopy images. The experiment was repeated in three independent donors with similar results. (e,f) Western blot analysis of lysates from sorted control and TNFi-exposed IL-17+ CD4+ T cells probed with mAbs against Aiolos or β-actin. A single blot (e) and cumulative data (mean with s.e.m.) quantified by densitometry (n=4. Normalized to actin by densitometry) (f) are shown. Full gels are shown inSupplementary Fig. 8. (g) Correlation betweenIKZF3andIL10expression in array samples (seeFig. 4for description), analysed by Pearson test. (h)IKZF3expression (normalized toPPIA, mean with s.e.m.,n=3) was measured by real-time PCR in sorted control or TNFi-exposed IL-17-IL-10- (Negs), IL-17+IL-10− (IL-17+), IL-17−IL-10+ (IL-10+) and IL-17+IL-10+ (dp+) CD4+ T cells. (i) Correlation betweenIKZF3andIL10expression in primary CD4+ T cells isolated from healthy donors as measured by real-time PCR (normalised toSDHA) and analysed by Pearson test. Figure 5: TNFi-exposed IL-17+ CD4+ T cells express increased levels of the transcription factor IKZF3 associated with IL10 expression. CD4+ T cells and monocytes were co-cultured with anti-CD3 mAb in the absence or presence of adalimumab, and IL-17+ CD4+ T cells were sorted on day 3. ( a ) The RMA-normalized expression intensity for IKZF3 is shown for n =9 paired samples (mean with s.e.m.). ( b ) IKZF3 expression (mean with s.e.m.) was determined in three independent samples by real-time PCR, normalized to GAPDH . ( c ) Confocal microscopy of sorted control and TNFi-exposed IL-17+ CD4+ T cells stained for Aiolos (green). Nuclei were stained with DAPI (blue). Inserts (right) show single cells, demonstrating co-localization of Aiolos with DAPI in both conditions. Scale bars, 40 μm; 10 μm in inserts. ( d ) Quantification (mean grey value with 95% CI, corrected for background) of Aiolos staining per nucleus from confocal microscopy images. The experiment was repeated in three independent donors with similar results. ( e , f ) Western blot analysis of lysates from sorted control and TNFi-exposed IL-17+ CD4+ T cells probed with mAbs against Aiolos or β-actin. A single blot ( e ) and cumulative data (mean with s.e.m.) quantified by densitometry ( n =4. Normalized to actin by densitometry) ( f ) are shown. Full gels are shown in Supplementary Fig. 8 . ( g ) Correlation between IKZF3 and IL10 expression in array samples (see Fig. 4 for description), analysed by Pearson test. ( h ) IKZF3 expression (normalized to PPIA , mean with s.e.m., n =3) was measured by real-time PCR in sorted control or TNFi-exposed IL-17-IL-10- (Negs), IL-17+IL-10− (IL-17+), IL-17−IL-10+ (IL-10+) and IL-17+IL-10+ (dp+) CD4+ T cells. ( i ) Correlation between IKZF3 and IL10 expression in primary CD4+ T cells isolated from healthy donors as measured by real-time PCR (normalised to SDHA ) and analysed by Pearson test. Full size image Expression of IKZF3 was found to correlate very strongly with IL10 expression in the array samples (Pearson’s test, r =0.89, P <0.0001) ( Fig. 5g ). To characterize which subpopulation of cells in the TNFi-exposed IL-17+ CD4+ T cell population expressed IKZF3 , we cultured CD4+ T cells and monocytes with anti-CD3 mAb in the absence or presence of adalimumab for 3 days and sorted CD4+ T cells based on IL-17 and/or IL-10 expression ( Supplementary Fig. 9 ). IKZF3 was expressed at the highest levels in the IL-10 expressing subsets (in both IL-10+IL-17− and IL-10+IL-17+ populations), and this was further enhanced following TNFi treatment ( Fig. 5h ). To further investigate the relationship between IL-10 and Aiolos, we measured the mRNA expression of their genes in freshly isolated primary CD4+ T cells from healthy donors, and found a strong correlation ( Fig. 5i ). Together these data suggested to us that the transcription factor Aiolos, encoded by IKZF3 , may be involved in the regulation of IL-10 expression in human CD4+ T cells. We wished to investigate whether Aiolos may also regulate IL-10 in IFN-γ+ CD4+ T cells (Th1 cells), because we found that these cells also showed an increase in IL-10+ cells following TNFi exposure ( Supplementary Fig. 10a,b ). In a similar approach as we had employed for IL-17+ CD4+ T cells, we cultured CD4+ T cells and monocytes with anti-CD3 mAb in the absence or presence of adalimumab. After 3 days we sorted the IFN-γ+ IL-17− CD4+ T cells and measured the expression of IKZF3 by qPCR and Aiolos by western blot. Although IKZF3 /Aiolos expression was increased in some individuals, overall we could not detect a consistent increase in TNFi-exposed Th1 cells ( Supplementary Figs 8 and 10c,d ). These data indicate to us that there is a strong relationship between Aiolos and IL-10 expression in IL-17+ CD4+ T cells, while this relationship is less consistent in IFN-γ+ CD4+ T cells. Aiolos drives IL10 in primary CD4+ effector T cells The strong association between IL10 and IKZF3 in IL-17+ CD4+ T cells suggested to us that Aiolos may play a role in the regulation of IL-10 expression in TNFi-exposed IL-17+ CD4+ T cells. To investigate this further, we first carried out an in-depth bioinformatical analysis of the IL10 genomic region ( Fig. 6a,b ). We found considerable evolutionary conservation in the IL10 locus and could detect five conserved putative Aiolos-binding sites (TGGGAA). Interestingly, all of these putative Aiolos-binding motifs are located either in the last intron or in the downstream region. To find out whether Aiolos interacts with these sites in TNFi-exposed IL-17+ CD4+ T cells, we employed chromatin IP (ChIP). Chromatin from TNFi-exposed IL-17+ CD4+ T cells was fragmented to 150–200 bp fragments, enabling us to distinguish between individual binding sites. We detected strong Aiolos binding to motifs in the last intron (motif 3), in the 3′ UTR (motif 4) and the downstream non-coding region (motif 5) ( Fig. 6c ). Of particular interest are motifs 4 and 5, which are located in narrow but evolutionarily ultraconserved regions, placed amidst diverged genomic territories ( Fig. 6a,b ). Conserved motifs 1 and 2, which are located in the 5′ end of the last intron, did not show significant Aiolos enrichment in our assay. The previously identified Ikaros-binding site in the IL10 promoter [20] demonstrated only a weak interaction with Aiolos. Overall, these data provide evidence for Aiolos binding to evolutionarily conserved regions in the last intron and downstream of IL10 . 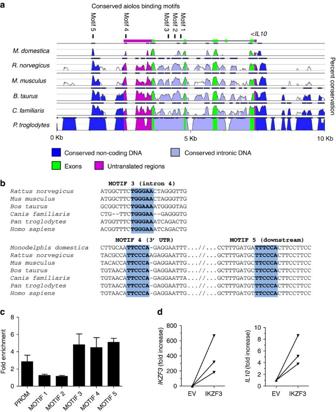Figure 6: Aiolos binds to theIL10genomic region in TNFi-exposed IL-17+ CD4+ T cells and drivesIL10expression in primary CD4+ effector T cells. (a) Analysis of sequence conservation in genomicIL10. Pair-wise sequence alignment to the human genome is depicted (50% lower cut-off), with evolutionarily conserved regions identified where identity above 70% over 100 bp was scored. These conserved genomic regions were searched for conserved consensus Aiolos DNA-binding motifs, shown at the top of the graph and numbered from 1–5. (b) Multiple sequence alignment of putative Aiolos motifs 3, 4 and 5. The consensus binding site is shown in bold and highlighted in blue. (c) ChIP-PCR of sorted TNFi-exposed IL-17+ CD4+ T cells shows Aiolos enrichment at motifs 3, 4 and 5. Analysed DNA motifs are demonstrated on the horizontal axes and numbered according toFig. 6a. PROM indicates the previously found Ikaros-binding sites in the promoter of mouseIL10.The values were normalized to two negative control regions (titin exons) to find enrichment of Aiolos binding at a region of interest over background signal (fold enrichment is shown±s.e.m.). (d) Memory CD4+ T cells were co-transfected with a CMV-eGFP reporter vector and either CMV-IKZF3 or CMV-empty vector (EV). At 48 h eGFP+ cells were sorted andIKZF3andIL10expression determined by real-time PCR (data normalized toSDHA, mean±s.e.m.,n=3). Figure 6: Aiolos binds to the IL10 genomic region in TNFi-exposed IL-17+ CD4+ T cells and drives IL10 expression in primary CD4+ effector T cells. ( a ) Analysis of sequence conservation in genomic IL10 . Pair-wise sequence alignment to the human genome is depicted (50% lower cut-off), with evolutionarily conserved regions identified where identity above 70% over 100 bp was scored. These conserved genomic regions were searched for conserved consensus Aiolos DNA-binding motifs, shown at the top of the graph and numbered from 1–5. ( b ) Multiple sequence alignment of putative Aiolos motifs 3, 4 and 5. The consensus binding site is shown in bold and highlighted in blue. ( c ) ChIP-PCR of sorted TNFi-exposed IL-17+ CD4+ T cells shows Aiolos enrichment at motifs 3, 4 and 5. Analysed DNA motifs are demonstrated on the horizontal axes and numbered according to Fig. 6a . PROM indicates the previously found Ikaros-binding sites in the promoter of mouse IL10. The values were normalized to two negative control regions (titin exons) to find enrichment of Aiolos binding at a region of interest over background signal (fold enrichment is shown±s.e.m.). ( d ) Memory CD4+ T cells were co-transfected with a CMV-eGFP reporter vector and either CMV-IKZF3 or CMV-empty vector (EV). At 48 h eGFP+ cells were sorted and IKZF3 and IL10 expression determined by real-time PCR (data normalized to SDHA , mean±s.e.m., n =3). Full size image Finally, to determine whether Aiolos is sufficient to drive IL10 expression, we co-transfected primary memory CD4+ T cells from healthy controls with constructs encoding eGFP and IKZF3 , and sorted the eGFP+ cells after 2 days. IL10 expression was increased in eGFP+ cells that were transfected with the IKZF3 construct as compared with the empty vector (EV) control ( Fig. 6d ). Together, these data suggest that Aiolos is a transcriptional regulator of IL-10 expression in human IL-17+ CD4+ T cells, and potentially in other T helper cells. Aiolos was identified in 1997 as the second member of the IKAROS family of zinc-finger transcription factors to which Ikaros, Helios, Eos and Pegasus belong [21] . Like other IKAROS gene family members, Aiolos has multiple isoforms and can control gene expression by interacting with other family members and different transcriptional regulators, including chromatin remodelling complex components [22] . Aiolos deficiency leads to alterations in B cells and increased levels of serum immunoglobulins and autoantibodies, B cell hyperproliferation and lymphomas [23] . Although T cell development in Aiolos-null animals appeared relatively unaffected, an increase in TCR-mediated proliferative responses in thymocytes and peripheral T cells, and an increased percentage of IFN-γ- or IL-2-producing peripheral T cells has been reported [23] . Recently, Quintana et al . [24] demonstrated that Aiolos silences the Il2 locus in mice, and that Aiolos-deficient mice show reduced Th17 and increased Th1 cell differentiation in vitro and in vivo . The authors suggested that Aiolos, through its repressive effects on Il2 transcription, promotes Th17 differentiation, consistent with previous observations that IL-2 inhibits Th17 differentiation in mice [25] . Whether IL-2 exerts similar inhibitory effects on human Th17 cell development is not firmly established; in fact, addition of IL-2 seems a prerequisite in human in vitro Th17 differentiation/expansion protocols [26] , [27] . Moreover, we found a small increase rather than a decrease in IL-2 in conditions where IKZF3 was increased ( Supplementary Fig. 11 ). An important difference between the study by Quintana et al . [24] and our study is that we observed the effects of Aiolos in effector CD4+ T cells, while Quintana et al . [24] studied the role of Aiolos in naive CD4+ T cell differentiation. Taken together, these findings suggest that Aiolos may affect CD4+ T helper cells differently depending on their differentiation stage. Our findings indicate that Aiolos may act as a direct transcriptional regulator of IL10 in CD4+ T cells. Using sorted TNFi-exposed IL-17+ CD4+ T cells, we show that Aiolos binds in the 3′ region of the IL10 locus. There is strong Aiolos binding to evolutionarily conserved regions with consensus motifs located 2,192 bp downstream of the STOP codon, 959 bp from the start of the 3′ UTR and 584 bp from the beginning of intron 4. Interestingly, analyses of large-scale chromatin modification and transcription factor–DNA interaction screens, made available by the ENCODE consortium [28] , [29] , demonstrate that our identified binding regions are possibly active in other cell types. For example, both intronic and downstream regions are covered by H3K27 acetylation signature, signifying an active, open state of chromatin [30] , [31] . The downstream region is also located in a DNase hypersensitivity cluster and occupied by p300, further suggesting transcription factor recruitment at this site [32] . Indeed, the ENCODE ChIP data on cultured cell lines illustrate binding of SP1 to intron 4 and the downstream conserved region of IL10 , and binding of MEF2A to these conserved genomic regions as well as to the 3′ UTR of IL10 . These two factors have previously been linked with IL10 transcriptional regulation [33] , [34] . Based on ENCODE data IRF4 binding could be detected in IL10 intron 4 and STAT3 binding in the downstream region. Both of these factors have also been associated with IL10 regulation in different cell types and conditions [35] , [36] , [37] . ENCODE results demonstrate NFκB binding in intron 4, the UTR and the downstream conserved region of IL10 . Finally, Ikaros can be bound at these conserved regions in lymphoblastoid cell lines [28] , [29] . Future efforts are needed to understand how many of the transcription factor–DNA binding events that were identified in cultured cell lines (ENCODE) occur in vivo in CD4+ T cells and how the different factors interact to fine-tune IL-10 expression and CD4+ T cell behaviour. Overall, the emerging evidence suggests that IL10 transcription relies on transcription factor recruitment to downstream enhancers. In addition to finding Aiolos binding regions in the IL10 locus we show here the functional consequence of this transcription factor recruitment, since IKZF3 overexpression was sufficient to drive IL10 expression in CD4+ T cells. IKAROS family members have been characterized mostly as transcriptional repressors [38] , [39] , [40] . Our results suggest a transcriptional activator function for Aiolos in CD4+ T cells. It is well established that IL-10 can be expressed by multiple CD4+ T cell subsets, supporting the concept that IL-10 functions as a negative regulator following immune cell activation [6] . IL-10 co-expression in Th1 cells can be mediated by various pathways including STAT4, ERK, c-MAF and Notch [6] , [41] . We observed that TNFi-exposed IFN-γ+ CD4+ T cells also showed an increase in the percentage of IL-10+ cells; however, this was not associated with a consistent upregulation of IKZF3 /Aiolos. It is possible that IL-10 regulation is differentially regulated in different Th subsets. We do not exclude the possibility however that Aiolos is involved in IL-10 regulation in cell types other than IL-17+ CD4+ T cells, as our data indicate that following TNFi exposure IKZF3 is increased in both IL-10+IL-17− and IL-10+IL-17+ cells. We also found that IKZF3 and IL10 expression are strongly correlated in primary CD4+ T cells ex vivo , and that IKZF3 overexpression results in increased IL10 expression in bulk memory CD4+ T cells. Together, our results suggest that increased expression of Aiolos in CD4+ T cells allows these cells to gain regulatory potential in the form of IL-10 production. In this regard, it is of interest to note that in the study by Quintana et al . [24] the upregulated Aiolos expression was found in Th17 cells that were differentiated in the presence of IL-6 and TGF-β1, a differentiation protocol that leads to the generation of non-pathogenic Th17 cells [9] , [10] , [24] . Indeed, Lee et al . [42] recently demonstrated that IKZF3 expression was part of the transcriptional signature of non-pathogenic Th17 cells. An immunoregulatory role of Aiolos is furthermore supported by reports that Aiolos is expressed in inducible Tregs [24] . IL-17 and IL-17+ CD4+ T cells are considered to be important contributors to synovial inflammation and bone erosion in experimental and clinical arthritis [3] , [43] , [44] , [45] , [46] , [47] . Although IL-17+ CD4+ T cells constitute a relatively small population in human blood, these cells are enriched in the inflamed joint and can have potent pro-inflammatory activity [3] , [43] , [48] . The acquisition of anti-inflammatory function through IL-10 expression by a substantial proportion of these cells may therefore aid in reducing inflammation. Although the IL-17+IL-10+ CD4+ T cell population is relatively small in size, studies in animal models have shown their potential in regulating inflammation, thus demonstrating their in vivo relevance [10] , [11] . Given that TNFi treatment promotes IL-10 expression not only in IL-17+ CD4+ T cells but also in IFN-γ+ T cells, and possibly other effector cells, the concerted increase in IL-10 production is likely to result in a less inflammatory environment. Our findings that IL-10+ CD4+ cells are increased following TNFi therapy in vitro and in vivo is in line with earlier work on mouse transgenic T cells and human tetanus-specific T-cell clones, which showed that chronic TNF exposure decreased IL-10 production while TNF blockade increased IL-10 (refs 49 , 50 ). Recently, several research groups have investigated the effect of TNFi treatment specifically on peripheral IL-17+ CD4+ T cells in vivo , with studies reporting increased [51] , [52] , [53] as well as decreased [54] percentages. The increase in peripheral IL-17+ CD4+ T cells was suggested to be due to impaired Th17 homing to the joint [52] . Our findings that TNFi drugs increase the percentage of IL-10+ cells within the IL-17+ CD4+ T population provides an additional explanation as to why an increase in IL-17+ CD4+ T cells does not necessarily lead to an increase in pathogenic potential and may therefore co-exist with successful TNFi therapy. Further large-scale studies are required to identify whether Aiolos is upregulated upon treatment in vivo and whether this can be linked to response, although a recent genome-wide association study of genetic predictors of TNFi treatment efficacy in RA did not identify IKZF3 as a significant locus [55] . It is interesting to note that the co-expression of IL-10 by IL-17+ CD4+ T cells in our in vitro studies could be blocked by the addition of the pro-inflammatory cytokine IL-1β. This finding corroborates a recent report that IL-1β can regulate IL-10 expression in human IL-17+ CD4+ T cells [12] , and suggests that depending on the inflammatory environment IL-17+ CD4+ T cells may be more or less pathogenic. In conclusion, our data provide further evidence for the intrinsic ability of CD4+ effector T cells to have regulatory activity through the expression of the anti-inflammatory cytokine IL-10. We demonstrate that TNF-α blockade results in increased IL-10 responses in human CD4+ T cells and propose a role for Aiolos as a transcriptional regulator of this process. Patient and healthy control samples Blood samples from patients with RA were obtained from the Rheumatology outpatient clinic at Guy’s Hospital. Disease activity score (DAS28), erythrocyte sedimentation rate, C-reactive protein, rheumatoid factor seropositivity, age, sex and disease duration were documented on the day of sample collection (see Supplementary Fig. 2 ). Healthy control samples were obtained from local healthy volunteers. Analysis of blood samples from patients with peripheral spondyloarthritis was performed on cryopreserved PBMC [13] . All clinical investigation was conducted according to Declaration of Helsinki principles. The work in this study was approved by the Bromley Research Ethics Committee and the local Ethics Committee of the AMC. Written informed consent was received from participants before their inclusion in the study. PBMC and cell subset isolation PBMC were isolated by density gradient centrifugation (Lymphocyte separation media, PAA, Pasching, Austria). Cell subsets were purified by magnetic cell separation according to the manufacturer’s instructions (Miltenyi Biotec, Bergisch-Gladbach, Germany) and purity was confirmed by flow cytometry. Monocytes (average purity >95%) were isolated by positive selection using anti-CD14 microbeads. CD4+ T cells were isolated via negative depletion resulting in an average purity of >99%. In some experiments, CD4+ T cells were separated into CD45RO− and CD45RO+ cells using CD45RO beads (average purities 97% and 89%, respectively). CD4+CD25− T cells (average purity 85% CD25−) were obtained by CD4+CD25+ T cell depletion using CD25 MicroBeads. Cell culture CD4+ T cells (0.5 × 10 6 ) and CD14+ monocytes (0.5 × 10 6 ) were co-cultured in 48-well plates in culture medium (RPMI-1640 (Gibco, Camarillo, CA, USA), supplemented with 1% penicillin/streptomycin, 1% L -glutamine (Gibco) and 10% heat-inactivated fetal calf serum (Sigma, UK), in the presence of 100 ng ml −1 anti-CD3 mAb (OKT3, Janssen-Cilag Ltd, High Wycombe, UK). The TNFi drugs infliximab (Janssen Biologics), adalimumab (Abbott), etanercept (Pfizer) and certolizumab (UCB Pharma) were purchased from Guy’s Hospital Pharmacy, prepared according to manufacturers’ instructions and frozen in aliquots at −20°C or kept at 4°C (certolizumab). All TNFi drugs were added in vitro at 1 μg ml −1 based on previous work [15] ; human IgG1 Fc (R&D Systems, UK) and human IgG1 (Abcam, UK) were added at the same concentration as TNFi drugs. In some experiments, anti-CD3/CD28 beads (Invitrogen, Paisley, UK) were added to T cells at a ratio of 0.2:1, or PBMC depleted of CD14+ monocytes and CD4+ T cells were added as accessory cells at a 1:1 ratio. Transwell experiments were performed using a 0.4 μm semi-permeable membrane insert (Corning). Where indicated, FcγR-blocking reagent (10 μl ml −1 , Miltenyi Biotec), blocking TNFRI/II Ab (5 μg ml −1 , R&D Systems), neutralizing anti-IL-10 mAb (clone 23,738, 10 μg ml −1 , R&D Systems), blocking IL-10R mAb (clone 37,607, 10 μg ml −1 , R&D Systems), hrTNF-α (10 ng ml −1 , R&D Systems) or hrIL-1β (10 ng ml −1 , R&D Systems) were added at the start of the co-culture. Functional characterization of IL-17-secreting cells CD4+ T cells and monocytes were co-cultured at a 2:1 ratio with anti-CD3 mAb ± adalimumab (1 μg ml −1 ). After 3 days, cells were stimulated with PMA (50 ng ml −1 , Sigma-Aldrich, St Louis, MO, USA) and ionomycin (750 ng ml −1 , Sigma-Aldrich) for 1.5 h, followed by an IL-17 and/or IL-10 cytokine secretion assay, or where indicated an IFN-γ secretion assay (Miltenyi Biotec), according to the manufacturer’s instructions. CD14− cells were sorted using a FACSAria II (BD, Franklin Lakes, NJ, USA) based on expression of IL-17-PE and/or IL-10-APC. Re-isolated total IL-17+ cells (20,000–200,000 cells) were stored in TRIzol (Invitrogen) for gene expression profiling or RNA was isolated using the RNeasy mini plus extraction kit (Qiagen, Germantown, MD, USA) for real-time PCR, or cells were cultured overnight in culture medium (100,000 cells per well) for cytokine secretion. In some experiments, IL-17+ cells (50,000 cells) were added to autologous or allogeneic CD14+ monocytes (100,000 cells) in the absence or presence of neutralizing anti-IL-10 mAb (10 μg ml −1 ) and monocyte phenotype was assessed after 40 h by flow cytometry. Flow cytometry For ex vivo analysis, 1–5 × 10 6 PBMC were cultured in 24-well plates for 3 h in the presence of PMA, ionomycin and GolgiStop (according to the manufacturer’s instructions; BD, Oxford, UK). Cells were stained for cell surface markers using CD3-PE-Cy7 (1:100) and CD14-APC-Cy7 (1:100) (BioLegend, Cambridge, UK), fixed in 2% paraformaldehyde, permeabilized with 0.5% Saponin and stained for CD4-PacificBlue (1:100) in combination with IL-17-PE (1:20), IFN-γ-PerCP-Cy5.5 (1:200), IL-10-AF488 (1:20) and TNF-α-APC (1:100) (all BioLegend). Co-cultures were re-stimulated at day 3 with PMA/ionomycin for 6 h, with GolgiStop present during the last 3 h. Cells were stained for cell surface markers using CD2-Pacific Blue (1:1,000) (BioLegend), CD14-APC-Cy7, fixed in 2% paraformaldehyde and permeabilized with 0.5% Saponin and stained for IL-17-PE, IFN-γ-PerCP-Cy5.5, IL-10-AF488 and TNF-α-APC. Foxp3 was measured using Foxp3-AF647 (1:20) (BioLegend) according to the manufacturer’s instructions. Monocyte phenotype was determined by staining with antibodies to CD14-APC-Cy7 (BioLegend), HLA-DR-PerCP-Cy5.5 (1:50) (BD), CD40-PE (1:50) (AbD Serotec, Kidlington, UK) and CD163-FITC (1:50) (Santa Cruz, Santa Cruz, CA, USA). Cells were acquired using a FACSCantoII (BD) and analysed using FlowJo software (TreeStar, Inc). Detection of soluble cytokines Monocyte/T cell co-culture supernatants were collected at day 3 after stimulation with PMA/ionomycin and stored at −80°C. Cytokine levels were determined by ELISA using R&D Systems DuoSets for IL-17A, IL-10 and IFN-γ according to the manufacturer’s instructions. Cytokine levels in supernatants from sorted IL-17-secreting T cells were determined using a Human Cytokine 25-Plex Panel (Invitrogen, Carlsbad, CA, USA) according to the manufacturer’s instructions. Gene expression profiling and analysis Sorted IL-17+ cell samples were lysed in 500 μl of TRIzol (Invitrogen). Chloroform (0.2 ml) was added to 1 ml TRIzol cell homogenate and whirl-mixed for 15 s. Homogenates were incubated for 2–3 min at RT and centrifuged for 15 min at 10,000 g (4 °C). The aqueous phase containing the RNA was further purified using RNeasy MinElute Cleanup Kit (Qiagen). RNA integrity was confirmed on an Agilent 2,100 Bioanalyzer using total RNA nano chips (Agilent Technologies, Santa Clara, CA, USA). An amount of 100 ng of total RNA was used to prepare targets by 3′ IVT Express kit (Affymetrix, Santa Clara, CA, USA) following the manufacturer’s instructions. Hybridization cocktails were hybridized onto Human Genome U133 Plus 2.0 GeneChips (Affymetrix) at 45°C for 17 h (60 r.p.m.) in a Hybridization Oven 640 (Affymetrix). GeneChips were washed and stained in a GeneChip fluidics station 450 using the fluidics protocol ‘EukGE-WS2v5_450’ (Affymetrix). Chips were scanned in a GeneChip scanner 3,000 (Affymetrix). Microarray data were normalized and gene expression measures derived using the RMA algorithm and the Bioconductor package ‘Affy’ ( http://www.bioconductor.org ). Custom CDF (chip definition file) from brainarray.mbni.med.umich.edu was used. Qlucore Omics Explorer 2.2 (Qlucore AB, Sweden) was used for the statistical analysis of the normalized data. Real-time PCR RNA was extracted with the RNeasy mini or RNeasy micro plus kit (Qiagen) and cDNA transcribed using a Reverse Transcription kit (High Capacity cDNA RT Kit, Applied Biosystems, Paisley, UK) according to the manufacturers’ instructions. Real-time PCR reactions were performed in multiple replicates and run on an ABI Prism 7900HT sequence detection system (Applied Biosystems) using a SYBR Green PCR mastermix (Applied Biosystems). All primers are listed in Supplementary Table 1 . Results were calculated using both the d C t method and the standard curve method and were normalized to two housekeeping genes. Confocal microscopy Control and TNFi-exposed IL-17+ CD4+ T cells were sorted and allowed to adhere onto poly- L -lysine-coated cover slips for 45 min at 37 °C. Cells were fixed with 4% PFA and permeabilized in the presence of triton X-100 (Sigma). Staining with rabbit anti-human Aiolos mAb (clone EPR9342(B), Epitomics, 1:10,000 dilution) (or an appropriate isotype control) was followed by incubation with goat anti-rabbit AF488 (Invitrogen) and DAPI (Invitrogen). Cover slips were mounted onto slides and slides imaged using an inverted Leica TCS SP5 DMI6000 confocal laser-scanning microscope (× 63 1.4NA oil immersion objective). To minimize fluorophore overlap DAPI stain (excited at 405 nm) and Aiolos (488 nm) were acquired sequentially. For quantification, Z projections (sum of slices) from eight fields of view were acquired for each condition and DAPI staining used to define a region of interest around the nucleus. Ten background measurements were collected per field and subtracted from the mean grey intensity of each cell measured. Western blotting Cells were washed with cold PBS followed by direct lysis in Laemmli buffer (Sigma-Aldrich). Lysates were boiled for 5 min at 95°C and resolved by electrophoresis using 4–12% Bis-Tris NuPAGE gels (Life Technologies Ltd, Paisley, UK). Proteins were transferred onto PVDF membranes (Merck Millipore, Billerica, MA, USA), which were cut horizontally near the 50 kD marker and probed with either anti-IKZF3 (1:5,000) (EPR9342(B), Epitomics) or anti-beta-actin (1:5,000) (13E5, Cell Signaling Technology, Danvers, MA), followed by horseradish peroxidase-conjugated polyclonal swine anti-rabbit immunoglobulins (1:3,333) (Dako, Glostrup, Denmark). Blots were developed with SuperSignal West Pico Substrate (Thermo Scientific, Rockford, IL, USA). Signals were acquired with the ChemiDoc XRS+ System using Image Lab software (Version 3.0, both Bio-Rad, Hemel Hempstead, UK) and quantified using ImageJ (Version 1.48b, NIH, Bethesda, MA). Chromatin immunoprecipitation TNFi-exposed IL-17+ CD4+ T cells (4 × 10 6 ) were sorted, washed in PBS, fixed at room temperature for 15 min in 1% formaldehyde and incubated 10 min in 0.125 M Glycine. Cells were washed 2 × in PBS, resuspended in 42 μl lysis buffer (100 mM NaCl, 50 mM Tris–HCl (pH 8.1), 5 mM EDTA, 1% SDS) and incubated on ice for 15 min. Dilution buffer (88 μl; 167 mM NaCl, 16.7 mM Tris–HCl (pH 8.1), 1.2 mM EDTA, 1.1% Triton X-100, 0.01% SDS) was added to lysis buffer and the sample was transferred to a Covaris microtube. Chromatin was sheared with Covaris E220 to achieve average fragment sizes between 150–200 bp. After chromatin shearing the sample was diluted further by dilution buffer (total volume 420 μl) and centrifuged at maximum speed to remove insoluble cell debris. Millipore Magna ChIP Protein A-G beads were blocked with blocking buffer (0.2 mg ml −1 glycogen, 0.2 mg ml −1 BSA, 0.2 mg ml −1 yeast RNA in dilution buffer) overnight at 4 °C. Sheared chromatin was precleared with blocked beads for 1 h at 4 °C and centrifuged at 13,000 g for 5 min, after which 10% of the sample was removed for input control. 400 μl of the precleared chromatin was transferred to a new tube to bind 3 μg of antibody on a rotating platform (6 h at 4 °C). After 15 min centrifugation at 13,000 g the antibody–chromatin solution was transferred to blocked magnetic beads and incubated overnight at 4 °C on a rotating platform. Next, the bead–DNA–antibody complex was washed twice in ChIP dilution buffer, once in low-salt buffer (standard ChIP buffer compositions), twice in high-salt buffer, once in LiCl buffer and twice in TE. Reverse crosslinking was carried out overnight at 65 °C and DNA purification was performed with IPure magnetic beads (Diagenode). qPCR for Aiolos enhancers and negative control regions was performed in duplicate with primers listed in Supplementary Table 1 . The efficiency of ChIP was estimated for each chromatin region as a percent from the total input chromatin sample. The values were normalized to two negative control regions (titin exons) to find enrichment of Aiolos binding at a region of interest over background signal (fold enrichment is shown ±s.e.m.). Transfection Primary memory CD4+ T cells from healthy donors were stimulated with 10 ng ml −1 PMA and 150 ng ml −1 ionomycin for 18–20 h. Cells were co-transfected with 5 μg cmv-eGFP and 5 μg p-CMV-SPORT-IKZF3 (IRATp970D0655D, Source BioScience LifeSciences) or 5 μg p-CMV-SPORT (made by excising IKZF3 from the p-CMV-SPORT-IKZF3 vector using Not1 and Sal1) using the Amaxa Human T Cell Nucleofector kit (Lonza), according to the manufacturer’s instructions. Cells were then cultured for 48 h followed by sorting of the GFP+ cells for qPCR. Viability post transfection was ~60%, and the transfection efficiency in viable cells was 11–30%. Statistical and bioinformatical analysis Statistical testing was performed with GraphPad 5.03 (GraphPad, San Diego, CA, USA). Data sets were tested for normality using the D’Agostino and Pearson omnibus normality test, followed by statistical significance testing using the appropriate statistical tests as indicated in the legends. Datasets with n values <8 were always tested non-parametrically. For analysis of the microarray data, for each gene, a paired t -test was performed to compare the expression levels between the conditions (Adalimumab and control), using Qlucore Omics Explorer 2.2 (Qlucore AB, Sweden). Adjusted P -values (or q -values) were computed using the Benjamini–Hochberg procedure. P -values <0.05 were considered to be statistically significant. Evolutionarily conserved regions (70% similarity over 100 bp) were identified with ECR Browser [56] aligned by Mulan and searched for conserved Aiolos motifs by multiTF [57] , [58] . How to cite this article: Evans, H. G. et al . TNF-α blockade induces IL-10 expression in human CD4+ T cells. Nat. Commun. 5:3199 doi: 10.1038/ncomms4199 (2014). Accession codes : The microarray data are deposited in Gene Expression Omnibus (GEO) with accession number GSE51540 .